Design of protein switches based on an ensemble model of allostery Switchable proteins that can be regulated through exogenous or endogenous inputs have a broad range of biotechnological and biomedical applications. Here we describe the design of switchable enzymes based on an ensemble allosteric model. First, we insert an enzyme domain into an effector-binding domain such that both domains remain functionally intact. Second, we induce the fusion to behave as a switch through the introduction of conditional conformational flexibility designed to increase the conformational entropy of the enzyme domain in a temperature- or pH-dependent fashion. We confirm the switching behaviour in vitro and in vivo . Structural and thermodynamic studies support the hypothesis that switching result from an increase in conformational entropy of the enzyme domain in the absence of effector. These results support the ensemble model of allostery and embody a strategy for the design of protein switches. The ability to design allosteric proteins or protein switches has many applications from basic science, to biosensors, to selective protein therapeutics [1] . While a handful of switch design strategies have met with some degree of success [2] , [3] , the design of switches for an application prescribed input signal (for example, effector and environmental conditions) and desired output function (for example, binding, catalysis, fluorescence and so on) remains a challenge. Previously, we pursued a directed evolution approach to switch design in which the switches are built from existing protein domains with the prerequisite effector-binding (input) and functional (output) domains [4] , [5] , [6] . We constructed libraries that explore the sequence space comprising insertions of one domain into the other, with or without circular permutation of the insert domain. We identified switches from these libraries via suitable screens or genetic selections. These studies taught us that switches are rare among the domain fusions that retain the output functionality. A key question is what do the switches possess that non-switch fusions lack? While biochemical and biophysical studies of our switches have provided some insights into this question [5] , [7] , [8] , [9] , [10] , we decided to pursue a complementary approach by designing switches based on an ensemble allosteric model (EAM), wherein sensitivity can be tuned by remodelling the energy landscape [11] . The allosteric regulation of protein function is central to essentially all aspects of cellular function. The phenomenological and structural models that have dominated the view of allostery have provided many insights [12] , [13] , [14] , [15] . However, recent studies have illuminated the importance of protein dynamics in allostery [11] , [16] , [17] , [18] , [19] , [20] , [21] , [22] , [23] , [24] , [25] and confirmed the predictions of Cooper and Dryden [26] that allostery can manifest in the absence of significant changes in the ground state structure of the protein [17] , [22] , [27] . The importance of conformational degeneracy in allostery is encompassed in the conformational EAM [28] , [29] , [30] . This model possesses the same characteristic of any ensemble model in that it posits that all possible conformations (or states) of a protein are populated according to their respective energies, and allosteric effectors remodel this landscape. The EAM [28] , [29] , [30] , however, also provides a vehicle for rationalizing the relationship between binding and conformational changes in each domain, and thus provides insight into the role of conformational degeneracy (that is, conformational entropy) in determining the overall allosteric effect. Allostery manifests, for example, from having the effector shift the ensemble from a set of states for which the ensemble-weighted average is less active to a set of states for which the ensemble-weighted average is more active by changing the relative stabilities of the different states. One way to achieve this is to have the ensemble in the absence of effector populating many states (especially less active ones) and have binding of the effector preferentially stabilize active states. This role for conformational entropy in allostery is central to the design of allosteric proteins described herein. In nature, protein flexibility has shown to be important for protein function [31] . In some cases, cold-adapted enzymes incorporate more glycine residues, which modulate functional activity by altering the flexibility of the native state or increasing the population of states that do not bind the substrate in the absence of that substrate [32] , [33] , [34] . Similarly, the substitution of glycines at sites distant from the active site of adenylate kinase affects its activity by selectively increasing the probability of locally unfolded states (and thus altering conformational entropy) without perturbing the structural properties of the native fold [19] . Based on these studies, we hypothesized that the appropriate introduction of conformational flexibility into non-switch fusion proteins could impose differential effects on the structural fluctuations on the output domain in the presence and absence of effector, and thereby confer switch properties to the fusion. Here, we design fusion proteins to possess switching behaviours via the introduction of linkers designed to increase the conformational entropy of the enzyme domain in a temperature- or pH-dependent fashion. We confirm the switching behavior with cellular and enzymatic assays, and we present structural and thermodynamic studies that support our hypothesis. The switches we create have multilevel control, requiring both a particular environmental condition (temperature or pH) and ligand for activation. Design of switches We have previously shown how protein switches can be constructed by fusing a ligand-binding domain and an enzyme such that the ligand acts as an effector regulating enzyme activity [4] , [6] . However, fusions that will exhibit switching are difficult to predict. Fusions that retain at least some enzymatic activity rarely possess effector regulation. We sought to develop a strategy to convert such non-switch fusion proteins into switches via control of local conformational entropy using engineered linkers possessing conditional conformational flexibility. We cast the problem in terms of an EAM [11] , [28] , [29] ( Fig. 1 ). We hypothesized that most enzymatically active fusions lack allostery because the enzymatically active states of the fusion are considerably more stable than the inactive states even in the absence of the effector ( Fig. 1b ). Thus, enzymatically active states of the fusion dominate the distribution of states with or without effector. For such a scenario, allostery could be established by remodelling the energy landscape such that the active states in the absence of ligand have similar or lower stabilities than the inactive states in the absence of ligand ( Fig. 1c ). We hypothesized that such an increase in conformational entropy in the enzyme domain could be achieved by the proper introduction of conformational flexibility in the protein. Since conformational flexibility can be externally controlled (for example, through temperature), the resulting switches would be expected to have multilevel control, requiring the induction of conformational flexibility for the switching property. 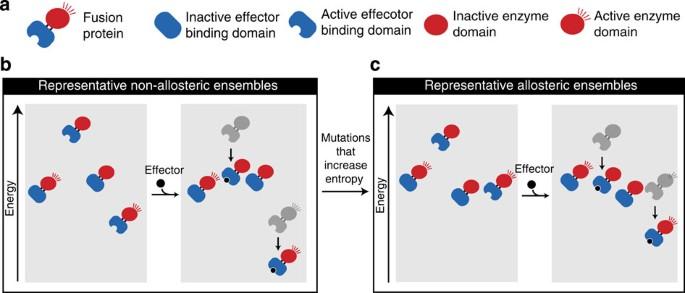Figure 1: Tuning an allosteric ensemble through mutations that promote conformational entropy. (a) The fusion proteins comprise two domains connected by two linkers (since one domain is inserted into the other). Each domain can be active or inactive (together with or separately from the other domain) resulting in four categories of representative states as shown. (b) Non-allosteric fusions lack allostery because states with an inactive enzyme domain are much less stable than states with an active enzyme domain regardless of the presence of ligand. (c) Allostery can be introduced though the introduction of conformational flexibility through mutation, where the flexibility increases the probability of the inactive states. Thus, the desired mutations remodel the energy landscape to increase the conformational entropy of the enzyme domain in the absence of ligand. The effector remodels the landscape by increasing the stability of states that bind the effector and thus their population in the ensemble, resulting in an effector-dependent increase in the observed enzyme activity. Although the schematic depicts the creation of positive allostery, negative allostery can be established in the same manner, as can be illustrated by switching the active and inactive domains in this figure (see Hilser and Thompson29). Figure 1: Tuning an allosteric ensemble through mutations that promote conformational entropy. ( a ) The fusion proteins comprise two domains connected by two linkers (since one domain is inserted into the other). Each domain can be active or inactive (together with or separately from the other domain) resulting in four categories of representative states as shown. ( b ) Non-allosteric fusions lack allostery because states with an inactive enzyme domain are much less stable than states with an active enzyme domain regardless of the presence of ligand. ( c ) Allostery can be introduced though the introduction of conformational flexibility through mutation, where the flexibility increases the probability of the inactive states. Thus, the desired mutations remodel the energy landscape to increase the conformational entropy of the enzyme domain in the absence of ligand. The effector remodels the landscape by increasing the stability of states that bind the effector and thus their population in the ensemble, resulting in an effector-dependent increase in the observed enzyme activity. Although the schematic depicts the creation of positive allostery, negative allostery can be established in the same manner, as can be illustrated by switching the active and inactive domains in this figure (see Hilser and Thompson [29] ). Full size image We chose to test this hypothesis for creating allostery using c4, a fusion protein between maltose-binding protein (MBP) and TEM1 β-lactamase (BLA), in which BLA is inserted into MBP in place of residues 317 and 318 of MBP, and is connected to residue 319 of MBP via a linker with the sequence DKT (ASP-LYS-THR) [9] ( Fig. 2a and Supplementary Table 1 ). c4 is not an allosteric protein and the c4 gene does not confer to Escherichia coli a maltose-dependent resistance to ampicillin (Amp) [10] . We reasoned that the introduction of conformational flexibility in the linker region of fusion proteins was most likely to cause the emergence of allostery in this fusion protein since the linker lies at the interface between the two domains ( Fig. 2b ). Furthermore, the introduction of changes in the linker minimized the chance of directly disrupting enzymatic activity or effector affinity. 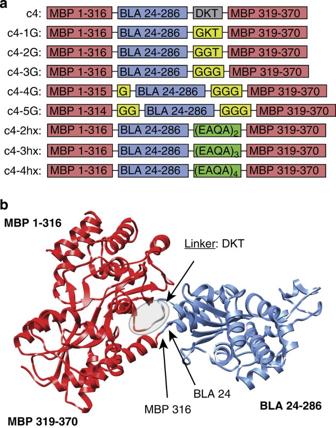Figure 2: Sequences and structural models of c4 and c4 variants. (a) Graphical illustration of the sequences of c4 and c4 variants indicating the MBP domain (red), BLA domain (blue), engineered glycine linker (yellow) and EAQA linker (green). (b) Structural model of the c4 fusion protein comprises MBP (red) and TEM-1 BLA (blue) domains with the DKT linker and fusion sites indicated by arrows. Figure 2: Sequences and structural models of c4 and c4 variants. ( a ) Graphical illustration of the sequences of c4 and c4 variants indicating the MBP domain (red), BLA domain (blue), engineered glycine linker (yellow) and EAQA linker (green). ( b ) Structural model of the c4 fusion protein comprises MBP (red) and TEM-1 BLA (blue) domains with the DKT linker and fusion sites indicated by arrows. Full size image We chose two methods to introduce flexibility: the substitution of glycines in the linker and the substitution of a peptide linker that undergoes pH-dependent conformational changes between α-helix and a random coil. Both of these methods afforded us non-mutagenic methods to control conformational entropy. Thus, we could interrogate the relationship between linker conformational flexibility and switching by changing the temperature for the glycine linker constructs and by changing pH for the pH-responsive linker constructs. This ability to control conformational entropy would result in multi-input switches, requiring the correct temperature or pH to be ‘turned on’ by the effector. pH-induced conformational conversion of (EAQA) n peptides Whereas the introduction of glycines was straightforward, the introduction of a peptide that would undergo pH-dependent conversion from an α-helix to a random coil required further design considerations. In previous studies, an amphipathic peptide was designed to interact with uncharged bilayers in a pH-dependent fashion through pH-induced random coil-α-helical transition [35] , [36] . We applied these design principles and chose an EAQA repeat peptide as a putative pH-responsive peptide ( Fig. 3a,b ). We designed the EAQA peptide to form an α-helix under acidic conditions. We positioned glutamate residues to align on one side of the helix so that they would destabilize the helix through charge repulsion at pH 7.5. 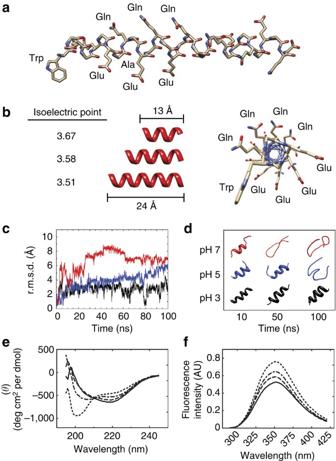Figure 3: Conformational conversion of the EAQA peptide. (a) α-Helical model of the WA-(EAQA)npeptide structure, (b) with isoelectric points and dimensions for two- to four-coiled α-helical structures: (EAQA)2–4and a cross-sectional view, showing side-chain residues. (c) MD simulation of the α-helical model of (EAQA)3peptide with increasing pH: pH 3 (black), pH 5 (blue) and pH 7 (red). Backbone r.m.s.d. relative to the initial structure as a function of simulation time at 300 K and (d) final structures after 10, 50 and 100-ns simulation. (e) CD spectra and (f) fluorescence emission spectra of WA-(EAQA)7at pH 4.5 (solid line), pH 5.5 (dashed line), pH 6.5 (dash-dotted line) and pH 7.5 (dotted lines). Figure 3: Conformational conversion of the EAQA peptide. ( a ) α-Helical model of the WA-(EAQA) n peptide structure, ( b ) with isoelectric points and dimensions for two- to four-coiled α-helical structures: (EAQA) 2–4 and a cross-sectional view, showing side-chain residues. ( c ) MD simulation of the α-helical model of (EAQA) 3 peptide with increasing pH: pH 3 (black), pH 5 (blue) and pH 7 (red). Backbone r.m.s.d. relative to the initial structure as a function of simulation time at 300 K and ( d ) final structures after 10, 50 and 100-ns simulation. ( e ) CD spectra and ( f ) fluorescence emission spectra of WA-(EAQA) 7 at pH 4.5 (solid line), pH 5.5 (dashed line), pH 6.5 (dash-dotted line) and pH 7.5 (dotted lines). Full size image We evaluated our design using structural modelling, molecular dynamic (MD) simulations and spectroscopic characterization. We conducted a 100-ns MD simulation using an α-helix model of the (EAQA) 3 peptide as a starting structure under three pH conditions: 3, 5 and 7 ( Fig. 3c,d ). Analysis of the positional root mean squared deviations of the backbone relative to the starting structure indicated that while the helix conformation at pH 3 remained relatively stable, the conformational conversion to random coil progressed as pH increased. We synthesized a 30-residue EAQA peptide, WA-(EAQA) 7 , that included a tryptophan at the N terminus and monitored the variation of its helical content by scanning the circular dichroism (CD) and tryptophan fluorescence spectra in solution at pH 4.5–7.5 ( Fig. 3e,f ). Ellipticity increased and fluorescence intensity decreased with increasing pH. Both findings are indicative of the desired α-helix to random coil structural change. We concluded that (EAQA) n peptides undergo a pH-dependent conversion from an α-helix to a random coil as designed. Designed proteins confer switch phenotype We constructed a series of variants of c4 in which one to three glycines were substituted into the DKT linker ( Fig. 2a ). In two constructs, glycines were also substituted at the other fusion point between the BLA and MBP domains. In addition, we created variants of c4 in which two to four repeats of the EAQA peptide replaced the DKT linker. We assayed for switching activity by measuring the minimum inhibitory concentration (MIC) for Amp for cells expressing these proteins in the presence and absence of maltose. We have previously shown that genes encoding MBP-BLA switches confer to E. coli cells a switching phenotype, that is, maltose-dependent resistance to Amp [5] , [9] , [10] . This phenotype arises from one or both of the following two mechanisms: maltose binding increases the specific Amp hydrolysis activity of the switch or maltose binding increases the cellular abundance of the switch, resulting in an increase in Amp hydrolysis activity in the cell [9] , [10] . Although the latter mechanism may not be classically thought of as allostery, it can be encompassed by a broader definition, as maltose modulates the properties of the protein in the cell. The switching phenotype is quantified by the fold increase in MIC afforded by the presence of maltose. For the glycine variants, we tested for a switching phenotype at both 18 and 37 °C. According to our hypothesis, switching should preferentially emerge at 37 °C. The progressive introduction of glycine residues (up to four glycines) monotonically increased the MIC Amp ratio to 32-fold at 37 °C, whereas no switching phenotype was observed at 18 °C ( Fig. 4a and Supplementary Tables 2 and 3 ). For the EAQA repeat variants, we tested for a switching phenotype at 37 °C on media at different initial pHs ranging from 6.0 to 8.0. The fusion proteins will experience these pH differences because they are expressed in the periplasm of E. coli . According to our hypothesis, switching should preferentially emerge at higher pH. We observed that the switching phenotype monotonically increased with pH and with the number of EAQA repeats, plateauing at three repeats and pH 8.0 with a 16-fold maltose-dependent switching phenotype ( Fig. 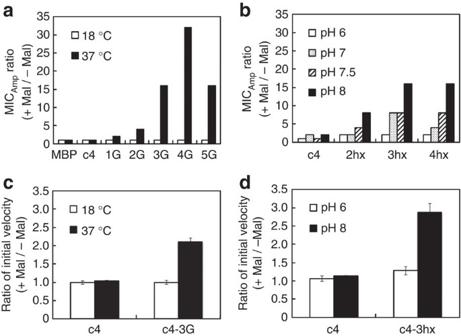Figure 4: Introduction of conformational flexibility results in cells with a switching phenotype and allosteric proteins. (a) Maltose-dependent fold increase in Amp resistance for cells expressing the indicated proteins at 18 and 37 °C. (b) Maltose-dependent fold increase in Amp resistance for cells expressing the indicated proteins grown in media with the indicated initial pH. The MICAmpratio (+maltose/−maltose) was calculated using the median MICAmpvalue from three independent trials. (c) Maltose-dependent fold increase in initial rate of nitrocefin hydrolysis enzymatic activity of c4 and c4-3G at 18 and 37 °C. (d) Maltose-dependent fold increase in initial rates of nitrocefin hydrolysis enzymatic activity of c4 and c4-3hx at pH 6 and 8, respectively. Average rates were calculated from three independent trials. 4b and Supplementary Table 4 ). In both sets of proteins, switching emerged as predicted by the model of Fig. 1 through a reduction in MIC in the absence of maltose. Figure 4: Introduction of conformational flexibility results in cells with a switching phenotype and allosteric proteins. ( a ) Maltose-dependent fold increase in Amp resistance for cells expressing the indicated proteins at 18 and 37 °C. ( b ) Maltose-dependent fold increase in Amp resistance for cells expressing the indicated proteins grown in media with the indicated initial pH. The MIC Amp ratio (+maltose/−maltose) was calculated using the median MIC Amp value from three independent trials. ( c ) Maltose-dependent fold increase in initial rate of nitrocefin hydrolysis enzymatic activity of c4 and c4-3G at 18 and 37 °C. ( d ) Maltose-dependent fold increase in initial rates of nitrocefin hydrolysis enzymatic activity of c4 and c4-3hx at pH 6 and 8, respectively. Average rates were calculated from three independent trials. Full size image Designed proteins are multi-input allosteric enzymes We purified c4 and c4-3G, and measured the rate of enzymatic hydrolysis of the BLA colorimetric substrate nitrocefin in the presence and absence of maltose at 18 and 37 °C ( Fig. 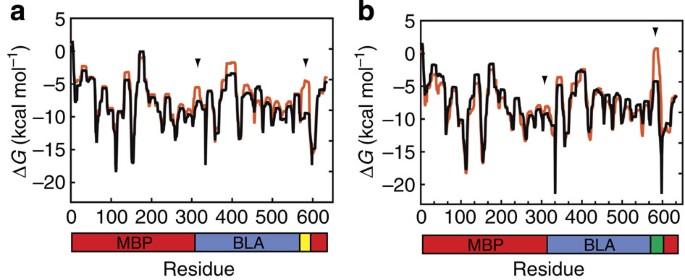Figure 5: Predicted residue stability using COREX/BEST. The predicted residue stabilities of (a) c4 (black) and c4-3G (red) and (b) c4-3hx in acidic (black) and basic (red) conditions are shown. These stabilities are based on the ratio of the summed probabilities of the states in the ensemble in which a particular residue is in a folded conformation to the summed probability of the states in which a residue is in an unfolded conformation. Arrowheads indicate fusion/linker sites. 4c and Supplementary Table 5 ). c4-3G’s catalytic activity depended on maltose at 37 °C but not at 18 °C. At 37 °C, the substitution of glycines in the linker of c4 established allostery by lowering the catalytic activity in the absence of maltose by 46% but decreasing the activity in the presence of maltose by only 12%, such that maltose increased catalytic activity twofold (2.05±0.15). At 18 °C, a temperature at which conformational flexibility of the linker is reduced, the introduction of glycines in the linker of c4 resulted in similar <10% decrease in catalytic activity in the presence and absence of maltose and no switching. The induction of switching by shifting the temperature to 37 °C was reversible, as shifting the temperature back to 18 °C resulted in the loss of the switching. Thus, the maltose-controlled switching property of c4-3G arises in temperature-dependent fashion, and c4-3G is a multi-input, allosteric switch. We compared the enzymatic activity of c4 and c4-3hx in the presence and absence of maltose at pH 6 and 8, respectively ( Fig. 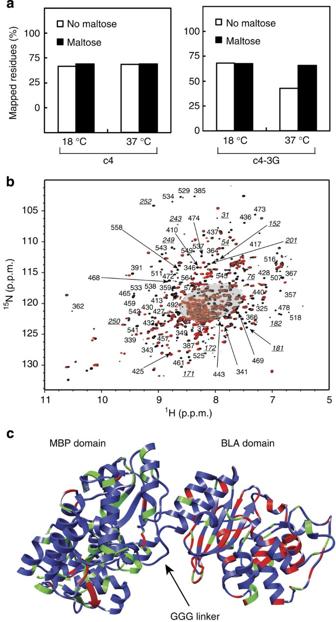Figure 6: Structural validation of protein switches. (a) Percentage of residues mapped from the15N-TROSY-HSQC spectra of c4 and c4-3G onto the spectra of MBP37and BLA38. (b) An overlay of the c4 (black) and c4-3G (red)15N-TROSY-HSQC spectra at 37 °C in the absence of maltose. The labels represent the peripheral peaks in the c4 spectrum that are not present in the c4-3G spectrum. These missing peaks were manually examined and attributed to residues of MBP (underlined italic) and BLA (regular text) domains. The central region of the spectra that was excluded from examination is shaded in grey. The corresponding missing residues are (c) mapped onto the MBP and BLA domain of the model structure of c4-3G and highlighted in red. Green indicates residues with peripheral resonances present in the spectra of both c4 and c4-3G. 4d and Supplementary Table 6 ). Only c4-3hx exhibited a maltose-dependent catalytic activity only at pH 8. At pH 6, the substitution of the pH-responsive (EAQA) 3 linker into c4 resulted in similar small increases in activity in the presence and absence of maltose and no switching. However, at pH 8, the introduction of the (EAQA) 3 linker reduced catalytic activity in the absence of maltose more than in the presence of maltose resulting in an approximately threefold (2.74±0.23) maltose-dependent increase in enzyme activity. The induction of switching by shifting the pH to 8 was reversible, as shifting the pH back to 6 by dialysis resulted in the loss of switching. Thus, c4-3hx is a multi-input, allosteric switch that requires the correct pH to exhibit switching. BLA domain experiences increased local structural entropy We next sought evidence that the switching properties of c4-3G and c4-3hx arose because the linker caused a change in the conformational entropy of the BLA domain in a temperature- and pH-dependent fashion, respectively. We constructed structural models of c4, c4-3G and c4-3hx, the latter both with the (EAQA) 3 peptide in helix and random coil form ( Supplementary Fig. 1 ). We analysed the effect of the new linkers on the local conformational entropy and stability using the ensemble-based structural thermodynamics algorithm COREX/BEST using these models. The algorithm predicted that substitution of the three glycines into c4 causes a significant decrease in stability near the fusion sites and an overall decrease in stability in the BLA domain ( Fig. 5a ). Conversion of the (EAQA) 3 peptide from helix form to random coil was predicted to reduced stability as well, but only in the (EAQA) 3 linker ( Fig. 5b ). Figure 5: Predicted residue stability using COREX/BEST. The predicted residue stabilities of ( a ) c4 (black) and c4-3G (red) and ( b ) c4-3hx in acidic (black) and basic (red) conditions are shown. These stabilities are based on the ratio of the summed probabilities of the states in the ensemble in which a particular residue is in a folded conformation to the summed probability of the states in which a residue is in an unfolded conformation. Arrowheads indicate fusion/linker sites. Full size image We next acquired [ 15 N and 1 H] TROSY-HSQC spectra (in the presence of deuteration) of c4 and c4-3G in the presence and absence of maltose at 18 and 37 °C, respectively. We compared these eight spectra with published chemical shift data of MBP [37] (BMRB 4,986 ligand free and BMRB 4,987 containing maltotriose) and BLA [38] (BMRB 6,357) as previously described [7] . The c4 and c4-3G spectra were consistent with the expectation that the individual domain structures were substantially conserved from MBP and BLA. As a quantification of this conservation of structure, we determined a peak count by counting peaks in the protein’s spectrum that appeared at the same location in the published peak assignments of BLA and MBP within a tolerance of ±0.2 p.p.m. on the 15 N axis and ±0.06 p.p.m. on the 1 H axis. About 55 peaks in the spectra of c4 and c4-3G did not have corresponding peaks in spectra of MBP or BLA, indicating that the residue may experience a different chemical environment than in the parental protein. Peaks present in spectra of the parental proteins but missing from the fusion proteins can result from the residue being in a different chemical environment, from peak broadening, resulting from the residue sampling a broader array of environments, and experimental limitations. Of the 634 residues of c4 and c4-3G, 579 residues had published peak assignments in the spectra of BLA [38] and MBP [37] . The peak counts of c4 and c4-3G (relative to those 579 potentially observable peaks) were very similar across all eight experiments (63–69%) with one exception ( Fig. 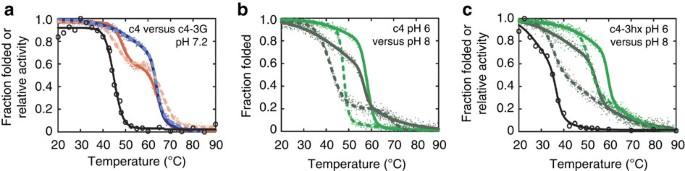Figure 7: Temperature unfolding of conformational switches. (a) Temperature unfolding transitions of c4 (solid red), c4 with 5 mM maltose (solid blue), c4-3G (dotted pink) and c4-3G with 5 mM maltose (dotted light blue) as assessed by the far-ultraviolet CD spectra at wavelength 222 nm. Open circles represent relative enzymatic activity of c4 as a function of temperature in the absence of maltose. Temperature unfolding transitions of (b) c4 and (c) c4-3hx in pH 6 (dotted green), pH 6 with 5 mM maltose (solid green), pH 8 (dotted dark green) and pH 8 with 5 mM maltose (solid dark green) as assessed by the far-ultraviolet CD spectra at wavelength 222 nm. Open circles represent relative enzymatic activity of c4-3hx as a function of temperature in the absence of maltose. 6a , Supplementary Figs 2–4 and Supplementary Table 7 ). The peak count of c4-3G in the absence of maltose at 37 °C was only 43%. We compared the c4 and c4-3G spectra resonances at 37 °C in the absence of maltose by overlaying the two spectra ( Fig. 6b ). Since the spectra for such a large protein is crowded near the centre, we focused our attention on resonances around the periphery ( Fig. 6b ) to reduce the frequency of misattributing resonances in the fusion protein in our mapping process. Although, some of these peripheral resonances may be misattributed in our process, the good match between resonances of c4 and the set of resonances of MBP and BLA suggests that most are correctly mapped, and that we can draw conclusions from the overall statistics. Of the 189 peripheral resonances mapped onto the sequence of c4, 107 were attribute to the MBP domain and 82 to the BLA domain. Seventy one of these 189 peaks were absent in the c4-3G spectrum ( Fig. 6b ). The BLA domain of c4-3G had much higher fraction of the absent peaks than the MBP domain (71 and 12%, respectively) ( Fig. 6c ). In addition, peaks throughout the entire BLA domain displayed broadening and low signal intensity for c4-3G at 37 °C in the absence of maltose ( Fig. 6b and Supplementary Fig. 2b ). Although this analysis is a selective examination of only residues with resonances in the periphery, this result is consistent with the BLA domain of c4-3G experiencing increased conformational entropy and flexibility only in the absence of maltose and only at 37 °C. Although similar selective broadening in fusion proteins might result from transient interactions between the domains or anisotropic tumbling, such effects would have to occur selectively in c4-3G at 37 °C in the absence of maltose for it to explain the lower peak count and resonance broadening under these conditions. Thus, these nuclear magnetic resonance (NMR) experiments provide good evidence that the introduction of conformational flexibility in the linker caused switch behavior through an increase in the conformational entropy of the BLA domain; however, more extensive NMR experiments will be necessary to solidify this interpretation. Figure 6: Structural validation of protein switches. ( a ) Percentage of residues mapped from the 15 N-TROSY-HSQC spectra of c4 and c4-3G onto the spectra of MBP [37] and BLA [38] . ( b ) An overlay of the c4 (black) and c4-3G (red) 15 N-TROSY-HSQC spectra at 37 °C in the absence of maltose. The labels represent the peripheral peaks in the c4 spectrum that are not present in the c4-3G spectrum. These missing peaks were manually examined and attributed to residues of MBP (underlined italic) and BLA (regular text) domains. The central region of the spectra that was excluded from examination is shaded in grey. The corresponding missing residues are ( c ) mapped onto the MBP and BLA domain of the model structure of c4-3G and highlighted in red. Green indicates residues with peripheral resonances present in the spectra of both c4 and c4-3G. Full size image We attempted to acquire NMR spectra of c4 and c4-3hx at 37 °C at pH 6 and pH 8; however, the proteins precipitated in solution. We were able to obtain spectra at 25 °C ( Supplementary Fig. 5 ). Most identifiable residues of c4 were also observed in c4-3hx. This indicates the preservation of structural integrity despite the replacement of the DKT linker with the relatively long and bulky (EAQA) 3 linker. No significant differences between the spectra of c4 and c4-3hx were apparent. 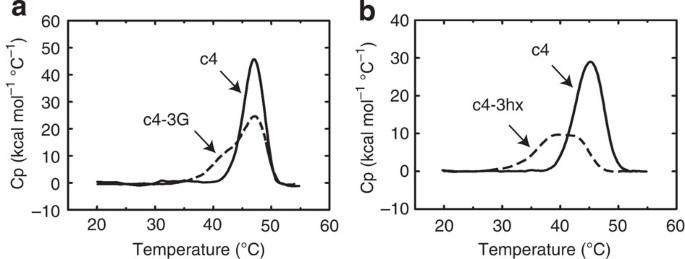Figure 8: Thermodynamic validation of protein switches. DSC thermograms in the absence of maltose for (a) c4 and c4-3G at pH 7.2, and (b) c4 and c4-3hx at pH 8. The thermograms shown correspond to the BLA domain and are representative of three independent experiments. Consistent with this result, we did not observe a switching phenotype when cells expressing c4-3hx were incubated at 25 °C ( Supplementary Table 8 ), unlike what we observed at 37 °C ( Fig. 4b ). Protein unfolding studies further supported the hypothesis that the introduction of conformational flexibility in the linker induced conformational heterogeneity in the BLA domain in the absence of maltose. In temperature-induced unfolding studies of c4 in the absence of maltose, the BLA domain unfolded reversibly at a lower temperature than the MBP domain with a transition midpoint ( T m ) slightly lower that reported for wild-type BLA [39] ( Fig. 7a and Supplementary Table 9 ). The addition of maltose shifted the unfolding of BLA to a higher temperature but rendered the unfolding irreversible. The substitution of the three glycines in c4 to create c4-3G decreased the T m of the BLA domain in the absence of maltose but not in the presence of maltose ( Fig. 7a and Supplementary Table 9 ). Similar to c4, the unfolding of the BLA domain of c4-3G was reversible only in the absence of maltose. Differential scanning calorimetry (DSC) experiments on the BLA domain in the absence of maltose revealed that the introduction of glycines in the linker caused the unfolding of the BLA domain to shift from a two-state, cooperative process to a non-two-state process with three possible unfolding domains ( Fig. 8a ), including one with a T m 4.5 °C lower than that of c4 ( Supplementary Table 10 ). Figure 7: Temperature unfolding of conformational switches. ( a ) Temperature unfolding transitions of c4 (solid red), c4 with 5 mM maltose (solid blue), c4-3G (dotted pink) and c4-3G with 5 mM maltose (dotted light blue) as assessed by the far-ultraviolet CD spectra at wavelength 222 nm. Open circles represent relative enzymatic activity of c4 as a function of temperature in the absence of maltose. Temperature unfolding transitions of ( b ) c4 and ( c ) c4-3hx in pH 6 (dotted green), pH 6 with 5 mM maltose (solid green), pH 8 (dotted dark green) and pH 8 with 5 mM maltose (solid dark green) as assessed by the far-ultraviolet CD spectra at wavelength 222 nm. Open circles represent relative enzymatic activity of c4-3hx as a function of temperature in the absence of maltose. Full size image Figure 8: Thermodynamic validation of protein switches. DSC thermograms in the absence of maltose for ( a ) c4 and c4-3G at pH 7.2, and ( b ) c4 and c4-3hx at pH 8. The thermograms shown correspond to the BLA domain and are representative of three independent experiments. Full size image We also conducted unfolding studies on c4 and c4-3hx at pH 6 and 8 ( Fig. 7b,c and Supplementary Table 9 ). Introduction of the pH-responsive linker into c4 had opposite effects on stability at the two pH values. Under conditions where the linker is more structurally ordered (pH 6.0), the introduction of the linker stabilized the protein, while at pH 8.0, when the linker is less ordered, the pH-responsive linker destabilized the protein. For c4-3hx, shifting the pH from 6.0 to 8.0 caused a much larger decrease in T m in the absence of maltose (−16.3±0.3 °C) than in the presence (−5.4±1.6 °C). DSC experiments at pH 8 on the BLA domain of c4 and c4-3hx in the absence of maltose mirrored that of c4 and c4-3G described above. The introduction of the linker caused a transition from two-state unfolding to non-two-state unfolding with unfolding domains with considerably lower T m values than that of c4 ( Fig. 8b and Supplementary Table 10 ), suggesting that multiple conformational states likely exist but with significantly lower stability. The EAM predicts that allostery can be established by remodelling the conformational ensemble through the introduction of conformational entropy in the absence of effector. We tested this prediction through the introduction of conformational flexibility in the linker region between a fusion of MBP and BLA. The resulting allosteric behavior of the proteins and the switch phenotype conferred to cells by the corresponding genes depended on the degree of conformational flexibility in the linker as modulated by linker composition or by environmental conditions (that is, temperature and pH). These results support our hypothesis in numerous ways on how the introduction of conformational flexibility can create allosteric switches. First, the introduction of conformational flexibility resulted in switch properties in vivo and in vitro . Second, switching depended on conformational flexibility, as reducing the temperature (for the glycine-substituted switches) or inducing helix formation by reducing the pH (for EAQA switches) eliminated the switching property. Third, switching arose as predicted by the model of Fig. 1 through a reduction in enzyme activity in the absence of maltose and not through an increase in enzyme activity in the presence of maltose. Fourth, the degree of switching monotonically increases with the degree of conformational flexibility introduced through the number of glycines or through the degree to which the pH-responsive peptide is expected to exhibit random coil behavior as controlled by pH. Fifth, biophysical studies support the hypothesis that linker flexibility induced an increase in the conformational heterogeneity of the BLA domain, which presumably allowed less-active states to be populated more frequently. Since we created allosteric proteins using two very different methods of introducing flexibility applied to the same fusion protein, the molecular details of how conformational flexibility is induced is not of primary concern. We propose that our approach potentially represents a general strategy for the introduction of allostery in non-allosteric proteins with the prerequisite effector-binding and functional properties. We note that the switches we created are multi-input switches, requiring a particular environmental condition (temperature or pH) and the presence of an effector (maltose) for activation. The 2–3-fold allosteric effect observed in vitro in our engineered proteins is comparable to the magnitude of effect in many natural allosteric enzymes. For example, E. coli aspartate transcarbamoylase, a classic example of an allosteric enzyme, exhibits only ∼ 4-fold changes in catalytic activity in the presence of saturating ATP and CTP [40] . Furthermore, the biological effect our switches provide to cells (up to 32-fold effect on the resistance phenotype) is certainly large enough to be relevant to cell engineering. We designed our proteins to have their switching property activated at a certain temperature or at a certain pH by the induction of disorder. Such activation has analogues in natural proteins. The yeast protein Hsp26 and the E. coli protein HdeA are chaperones that function to help the cell alleviate the negative effects of high temperature and low pH, respectively. Hsp26 is activated by an increase in the temperature [41] , and this activation is characterized by a decrease in ordered secondary structure [42] . HdeA shifts from its inactive, well-folded dimer to its active, partially unfolded monomer upon exposure to low pH [43] . Our approach in inducing allostery is counterintuitive from a mechanical/structural view of allostery. From that viewpoint, increased linker flexibility might be expected to decouple or dampen the transmittal of the signal from one domain to the other. However, theoretical [28] , [29] and empirical [44] , [45] studies have shown that allostery can be a property of proteins with intrinsically disordered domains. Thus, a structured linker is neither necessary nor sufficient for signal transmission. Whereas the aforementioned studies show that proteins with intrinsically disordered domains can possess allosteric properties, our experiments demonstrate something different. Our experiments demonstrate that allostery can emerge from the introduction of short, unstructured protein segments at the interface between two domains. In so doing, our work adds to the growing appreciation of how intrinsically disordered regions can contribute to protein function. Materials All chemicals used were purchased from Sigma (St Louis, MO) unless otherwise noted. NMR tubes were purchased from Shigemi (Allison Park, PA). Nitrocefin was purchased from EMD Millipore (Billerica, MA). BL21-competent cells were purchased from Agilent Technologies. Plasmids pDIMC8-c4h and pDIMC8-MBP that contain the c4 and malE genes, respectively, were previously described [9] , [10] . Plasmid pDIMC8-c4h was used as a template plasmid DNA to make linker variants using the PCR-based QuikChange mutagenesis procedure (Agilent Technologies). DNA sequencing of 2,013–2,061 bp regions containing the targeted codon confirmed mutant clones (Genewiz). The WA-(EAQA) 7 peptide (sequence: WAEAQAEAQAEAQAEAQAEAQAEAQAEAQA) was custom synthesized with 98% purity by Peptide 2.0.synthesis, and peptide ends were modified by N-terminal acetylation and C-terminal amidation. Molecular modeling and simulation The molecular models of c4 and the c4 variants were constructed with the amino-acid sequence and coordinates of MBP (PDB ID: 1OMP) and BLA (PDB ID: 1M40), and the distance constraints of the engineered MBP-BLA fusion protein, RG13 (PDB ID: 4DXC), using MODELLER software [46] . The sequence of residues 1–316 and 319–370 of MBP and residues 26–290 of BLA were aligned with the sequence of RG13, and the initial model of c4 was built using RG13 as a template. Since there was no structural information about the linker between the MBP and BLA domains, intermolecular distance between two domain obtained from RG13 were used as constraints to construct the initial models, and then ab initio loop optimization methods were used to model the linkers between residues 313 and 323 and 575 and 585. The linker-optimized model was then used as a template to optimize the model of c4 by repeating the steps described above. For c4-3G model, the amino-acid residues 580–582 were replaced with three glycine residues. For c4-3hx model, the residues 580–582 were replaced with a three-coiled α-helix and random coil structure model of the (EAQA) 3 peptide. The three-coiled α-helix model of EAQA (3hx) was built using UCSF Chimera [47] , and the random coil model was the final structure of the (EAQA) 3 model after 100 ns of MD simulation at pH 7 (described below). The model-building step was then repeated again with the (EAQA) 3 inserted models as templates to optimize the intermolecular distance between domains. The side-chain positions of the c4 and c4 variant models were subsequently optimized by using SCWRL 4.1 (ref. 48 ), and the final models were optimized by energy minimization using the GROMACS 4.1.3 package [49] . COREX/BEST [50] was used for statistical thermodynamic analysis of the c4 and c4 variant structure models at 37 °C. The model structures were used as templates to generate >10 5 partially unfolded states using Monte Carlo sampling strategy with the assumption that folded regions maintain native-like geometry and unfolded regions are modelled as fully solvated [16] . Folding units were defined by assigning sequential residues to different folding units (11 residues per unit), and different states were enumerated by folding and unfolding each unit. Folding units were varied by sliding the boundaries by one-residue increments and repeating the enumeration. The free energy of each state was determined using a surface area-based parameterization of the energetic. Each of c4 and c4 variant model was then characterized with the residue stability constant and relative free energy, which were calculated from the ratio of the summed probabilities of the states in the enumerated protein ensembles in which a particular residue is in a folded conformation to the summed probability of the states in which a residue was in an unfolded conformation [16] , [50] . MD simulations of EAQA peptide All simulations of (EAQA) 3 peptide were performed with the GROMACS software package [49] using the GROMMOS 43a3 force field [51] . The model structures used in the simulations were the simple α-helix model of (EAQA) 3 peptide. Simple EAQA models were solvated individually in octahedron boxes filled with water molecules [52] . A single-point charge water model was used for the solvent molecules in the simulation [53] . Sodium ions were used to electroneutralize the system. Solutes, solvent and counterions were coupled independently to reference temperature baths at 300 K (ref. 54 ), and the pressure was maintained by coupling the system weakly to an external pressure bath at 1 atm. Bond lengths were constrained by the LINCS procedure [55] and non-bonded interactions were evaluated using twin-range cutoff of 0.8 and 1.4 nm for Lennard–Jones and Coulomb potentials. The long-range electrostatic interactions beyond the cutoff were treated with the generalized reaction field model by using a dielectric constant of 54. The integration time step was set to 0.002 ps and the trajectory coordinates and energies were stored at 0.5 ps intervals. The analysis was performed using the built-in programs of GROMACS software package. To emulate the different pH environment, glutamate residues and the C terminus were protonated accordingly. Analysis was performed using the built-in programs of the GROMACS software package [49] . Expression and purification Proteins were expressed and purified from BL21 cells grown in M9 minimal media containing ammonium chloride (18.5 mM), thiamine (30 μM), MgSO 4 (2 mM), CaCl 2 (100 μM), fructose (50 mM), 2% glycerol (w/v) and chloramphenicol (50 μg ml −1 ). For production of each protein, 1 l of minimal media was inoculated with 10 ml overnight culture of BL21 cells, harbouring the pDIMC8 plasmid encoding the proteins, and shaken at 37 °C until the OD 600 reached 0.7. The culture was induced with 1 mM isopropyl-β-D-thiogalactopyranoside (IPTG) and incubated at 25 °C for another 48–50 h. For NMR study, proteins were prepared from M9/D 2 O minimal media containing 25 mM deuterated glucose-d7 (25 mM) and 15 NH 4 Cl (18.5 mM) as described in the previous study [7] . For production of labelled proteins in 1 l minimal media, a 10-ml overnight culture was prepared in lysogeny broth (LB)-rich media at 37 °C. The cells were then pelleted, washed and resuspended in 1 ml of D 2 O. The resuspension was diluted to 10 ml of labelled M9/D 2 O minimal media and grown overnight at 37 °C. The overnight culture was diluted to 100 ml with labelled M9/D 2 O minimal media and shaken at 37 °C. Once the OD 600 reached between 0.7, the cells were transferred to 2 l flask and diluted again to 1 l of labelled M9/D 2 O minimal media. The 1-l culture was incubated at 37 °C until the OD 600 reached 0.7, at which time IPTG was added to the culture to a final concentration of 1 mM to induce the proteins of interest. The 1 l culture was switched to a 25-°C shaker for 72 h. After expression, the cells were harvested and resuspended in 10 ml buffer (50 mM sodium phosphate and 150 mM NaCl, pH 7.2) and lysed using a French press. Cell lysates were centrifuged at 20,000 g for 1 h. The soluble proteins were purified using the HisTrap (GE Healthcare Life Sciences) and size-exclusion column in the AKTA FPLC purifier system (GE Healthcare Life Sciences). Proteins were dialysed against 15 l of a dialysis buffer (25 mM phosphate, pH 7.2) and concentrated using Amicon centrifugal filter (Millipore). For the NMR study, NaN 3 was added to 0.05%. Approximately 12 mg of purified proteins were obtained with >95% purity, estimated by Coomassie blue staining of SDS–PAGE gels. Protein concentration was determined using a NanoDrop spectrophotometer (Thermo Scientific) by measuring ultraviolet absorbance at 280 nm. Nitrocefin hydrolysis enzymatic assay Enzymatic assays were performed as previously described [9] , [10] Proteins were added to 100 mM sodium phosphate buffer, pH 7.2, to the final concentration of 1–5 nM, and were incubated in the absence and presence of 5 mM maltose for 5–30 min at 18 and 37 °C. For pH experiment, c4 and c4-3hx were incubated in pH-adjusted phosphate buffer (pH 6 and 8) for 30 min before the incubation with maltose. Nitrocefin was added to the final concentration of 100 μM. The absorbance at the wavelength of 486 nm was recorded by using a Varian Cary 50 UV-Visible Spectrophotometer (Agilent Technologies) and the initial rate of nitrocefin hydrolysis reaction was measured by Cary WinUV software package. MIC Amp assay For c4 and the c4 variants, the MIC Amp assay was performed as previously described [9] , [10] . BL21 cells were transformed with pDIMC8 plasmids containing genes that encode the protein variants. For each overnight culture, 5 ml of tryptone broth (10 g l −1 tryptone and 10 g l −1 NaCl) was inoculated by picking a single colony and incubated in a 37-°C shaker for 16–18 h. The optical density at 600 nm (OD 600nm ) was measured. For the MIC Amp assay, ∼ 1 × 10 6 colony-forming units (based on OD 600nm ) from the overnight culture were added to 1 or 5 ml of tryptone medium containing chloramphenicol (50 μg ml −1 ), IPTG (300 μM), Amp (0–8,192 μg ml −1 ), and either the absence or presence of 5 mM maltose in each culture tube. For temperature-dependent MIC Amp assay, 5 ml cultures were incubated in 18 and 37 °C shaker incubators for 36 and 18 h, respectively, and the OD 600nm of each culture was measured. For pH-dependent MIC Amp assay, pH of the tryptone medium was adjusted with HCl and NaOH, and 1 ml cultures in 96-well assay block (Corning, Tewksbury, MA) were incubated in 37 °C shaker incubators for 18 h. No growth was observed at pH 5. The MIC Amp was defined as the lowest concentration of Amp at which the OD 600nm was <5% of the OD 600nm in the absence of Amp. CD and fluorescence spectroscopy CD and fluorescence emission spectra of the WA-(EAQA) 7 peptide was scanned at 23 °C as previously described [35] . The WA-(EAQA) 7 peptide was dissolved in 50 mM TES at pH 7.5 (0.5 mg ml −1 ). The stock solution was diluted in a 5-mM 2-[[1,3-dihydroxy-2-(hydroxymethyl)propan-2-yl]amino]ethanesulfonic acid (TES)/100 mM KCl, with varying pH by NaOH and HCl, and incubated for 30 min before the scan. The far-ultraviolet CD spectra were recorded in a Jasco J-710 CD Spectropolarimeter (Jasco, Easton, MD), averaged over three scans at a spectral bandwidth of 1 nm with 2 s integration time using a quartz optical cell with an optical pathlength of 1 mm (Fisher Scientific). Fluorescence emission spectra were recorded in a PTI Quantamaster 30 Fluorescence Spectrofluorometer (Photon Technology International) with excitation at 280 nm and spectral bandwidths of 2 nm (excitation) and 4 nm (emission) using quartz cuvette (pathlength of 10 mm). The final concentration was 0.05 mg ml −1 for CD spectra and 0.005 mg ml −1 for fluorescence emission spectra. For c4 and c4 variants, thermal denaturation was examined by monitoring the far-ultraviolet CD spectra. Protein samples were incubated in the absence and presence of 5 mM maltose for 1 h at 4 °C in 50 mM phosphate buffer (pH 7.2) before thermal denaturation. To obtain the CD spectra at varying pH, the proteins were prepared in pH-adjusted 50 mM phosphate buffer (pH 6 and 8) before the incubation. The final protein concentration was 5 μM. CD absorbance at 222 nm was collected from 20 to 90 °C at a temperature ramp rate of 1 °C min −1 and a bandwidth of 1 nm. All spectra were buffer corrected. The data were normalized and fitted to a two-state and three-state unfolding model using Prism analysis software (GraphPad, La Jolla, CA). Differential scanning calorimetry For the calorimetric study of protein unfolding, the protein samples were dialysed overnight against a buffer containing 50 mM sodium phosphate and 5% w/v glycerol at pH 7.2 and 8, which was also used in the reference cell and for baseline determination. The final protein concentrations were 1 mg ml −1 . Heat absorbance was collected from 20 to 55 °C in a MicroCal VP-DSC instrument at a temperature ramp rate of 1 °C min −1 . Thermograms were baseline corrected, normalized and analysed according to two-state and non-two-state models with a single and multiple transitions, in which T m , Δ H cal and Δ H vH , and Δ C p of individual transitions were fitted independently using the MicroCal Origin software (Microcal, Northhampton, MA). NMR spectral acquisition Acquisition of TROSY-HSQC spectra was conducted as previously described [7] . D 2 O was added to 10% to a 200-μM sample of c4 and c4 variants. The 350 μl samples were then loaded into a Shigemi tube. Data were acquired on an 800-MHz ( 1 H) Varian INOVA spectrometer equipped with a cryogenic probe and z axis gradients at appropriate temperatures (18, 25 and 37 °C) in the presence and absence of 5 mM maltose. A sensitivity-enhanced TROSY sequence [56] was used, with 16 scans/FID and an interscan delay of 1.9 s. Spectral widths of 16 kHz ( 1 H) and 2,836 Hz ( 15 N) were used, with an acquisition time of 60 ms in both 1 H and 15 N dimensions. The total data collection time was 3.25 h per spectrum. Quadrature detection in the 15 N dimension was achieved using the echo–antiecho method [57] . The data were apodized with 60° phase-shifted cosine-squared bell window functions in both dimensions and zero-filled to a final digital resolution of 4 Hz pt −1 in 1 H and 1.4 Hz pt −1 in 15 N. Data were processed and analysed using NMRPipe and NMRView software (One Moon Scientific, Westfield, NJ). How to cite this article: Choi, J.H. et al . Design of protein switches based on an ensemble model of allostery. Nat. Commun. 6:6968 doi: 10.1038/ncomms7968 (2015).